Substrate stress relaxation regulates cell spreading Studies of cellular mechanotransduction have converged upon the idea that cells sense extracellular matrix (ECM) elasticity by gauging resistance to the traction forces they exert on the ECM. However, these studies typically utilize purely elastic materials as substrates, whereas physiological ECMs are viscoelastic, and exhibit stress relaxation, so that cellular traction forces exerted by cells remodel the ECM. Here we investigate the influence of ECM stress relaxation on cell behaviour through computational modelling and cellular experiments. Surprisingly, both our computational model and experiments find that spreading for cells cultured on soft substrates that exhibit stress relaxation is greater than cells spreading on elastic substrates of the same modulus, but similar to that of cells spreading on stiffer elastic substrates. These findings challenge the current view of how cells sense and respond to the ECM. Mechanical properties of extracellular matrices (ECMs) are thought to play an important role in regulating cell behaviours in development, tissue homeostasis and disease [1] , [2] , [3] , [4] , [5] . Studies investigating the influence of substrate elasticity on biological processes typically utilize two-dimensional (2D) surfaces of collagen or fibronectin-coated polyacrylamide gels as substrates for cell culture. These studies have found that cell spreading [6] , [7] , proliferation [8] and nuclear localization of the transcriptional regulator YAP (Yes-associated protein) [9] are all suppressed on soft substrates. The mechanistic understanding is that cells sense substrate elasticity by gauging resistance to the traction forces the cells exert on the substrate [10] , [11] . However, the covalent crosslinking of these polyacrylamide hydrogels results in purely elastic substrates with a time-independent storage or elastic modulus [12] . Correspondingly, deformations of the polymer matrix are elastic, not plastic, so that resistance to traction forces exerted by cells is constant over time, and elastic energy is stored in the substrate [13] . In contrast, reconstituted extracellular matrices, such as collagen [14] , or fibrin [15] , and many tissues [16] , [17] , [18] , exhibit stress relaxation, or a decrease in the storage or elastic modulus over time when a constant strain is applied. On such matrices, the resistance to cellular traction forces is expected to be relaxed over time due to flow and remodelling of the matrix, dissipating the energy that cell-generated forces imparted into the material. While broadly presented to cells under physiological conditions, the influence of substrate stress relaxation on cell behaviour is unknown. Here we investigate the role of substrate stress relaxation on cell spreading. First, computational modelling predicts that cell spreading is enhanced for cells adhering to viscoelastic substrates that exhibit stress relaxation relative to elastic substrates at low initial elastic moduli and high ligand densities. Next, cell-spreading experiments using purely elastic or viscoelastic alginate hydrogels as cell adhesion substrates confirm these predictions, finding that cells even spread on soft viscoelastic substrates to a similar extent as cells spread on stiffer elastic substrates. These results challenge the current view that cells sense ECM elasticity simply by gauging resistance to the traction forces they exert on the ECM Model predicts the impact of stress relaxation on cell spreading We first adapted a published model to predict the impact of stress relaxation on cell spreading. Since the time-dependent elastic modulus of substrates with stress relaxation decreases over time when strained by cell traction forces, the intuitive expectation is that cells would integrate the modulus over time, and thus respond to substrates with stress relaxation as if they were substrates with an effectively lower elastic modulus. If this were the case, cell spreading would be attenuated in all cases on substrates with stress relaxation relative to elastic substrates, given the same initial elastic modulus. A simple stochastic lattice spring model was developed to test this intuitive expectation on the very early stages of cell spreading ( Fig. 1a , Supplementary Note 1 , Supplementary Fig. 1 ). Following a recent model of filopodial protrusion [19] , [20] , this model considered cell spreading to be driven by polymerization of actin that was coupled to the surface of a substrate through molecular clutch adhesions, the key parameters relevant to the early stages of cell spreading, but additionally incorporated substrate stress relaxation and cell adhesion ligand density ( Fig. 1a ). The substrate was modelled as a series of nodes connected by either Hookean springs, representing an elastic substrate, or four-element Burgers models, representing a viscoelastic substrate that exhibits stress relaxation. Simulations of cell spreading on the basis of this model were run on either elastic substrates or substrates with stress relaxation, and the cell-spreading area was predicted as a function of cell adhesion-ligand density and initial stiffness ( Fig. 1b,c ). On both types of substrates, cell spreading increased as a function of stiffness, consistent with previous experimental findings. At high stiffness, the model predicts only small differences in spreading between elastic and relaxing substrates. Surprisingly though, the simulations reveal a regime, at low stiffness and higher ligand densities, in which cell spreading can be significantly enhanced on substrates with stress relaxation relative to elastic substrates ( Fig. 1d ), counter to the intuitive expectation. In the limit when the Burgers element becomes either a Maxwell element or a Voigt element, we find that the enhanced cell spreading on substrates that exhibit stress relaxation is better predicted in the case of the Voigt element ( Supplementary Fig. 2 ). While this model does not consider longer timescales and more complex feedback mechanisms [21] , it predicts an essential effect of substrate viscoelasticity when cells bind to substrates through molecular clutches. 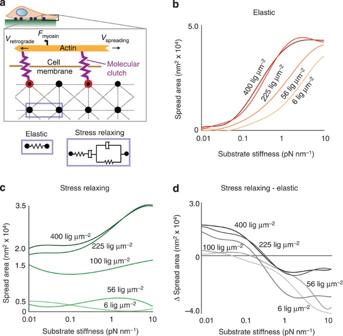Figure 1: Stochastic lattice spring model predicts increased cell spreading at low initial stiffness on viscoelastic substrates that exhibit stress relaxation relative to elastic substrates. (a) Schematic depicting model of cell spreading on elastic or viscoelastic substrates. Actin polymerization at the leading edge of the cell is coupled to the substrate through molecular clutches, and these clutches inhibit retrograde flow of the actin driven by myosin motors. The substrate is modelled as an array of nodes connected by either Hookean springs, representing an elastic substrate, or Burgers model elements, representing a viscoelastic substrate exhibiting stress relaxation. (b) Simulation results for the cell-spreading area on elastic substrates as a function of initial substrate stiffness and adhesion ligand density. (c) Simulation results for the cell-spreading area on substrates with stress relaxation as a function of initial substrate stiffness and adhesion ligand density. Voigt damping coefficient,η1, was 5 × 10−13, and Maxwell damping coefficient,η2, was 1 × 10−13for this set of simulations (SeeSupplementary Information). (d) Difference in the cell-spreading area for cells on substrates with stress relaxation relative to elastic substrates. Greater spreading on substrates with stress relaxation is observed for all conditions at low substrate stiffness. Figure 1: Stochastic lattice spring model predicts increased cell spreading at low initial stiffness on viscoelastic substrates that exhibit stress relaxation relative to elastic substrates. ( a ) Schematic depicting model of cell spreading on elastic or viscoelastic substrates. Actin polymerization at the leading edge of the cell is coupled to the substrate through molecular clutches, and these clutches inhibit retrograde flow of the actin driven by myosin motors. The substrate is modelled as an array of nodes connected by either Hookean springs, representing an elastic substrate, or Burgers model elements, representing a viscoelastic substrate exhibiting stress relaxation. ( b ) Simulation results for the cell-spreading area on elastic substrates as a function of initial substrate stiffness and adhesion ligand density. ( c ) Simulation results for the cell-spreading area on substrates with stress relaxation as a function of initial substrate stiffness and adhesion ligand density. Voigt damping coefficient, η 1 , was 5 × 10 −13 , and Maxwell damping coefficient, η 2 , was 1 × 10 −13 for this set of simulations (See Supplementary Information ). ( d ) Difference in the cell-spreading area for cells on substrates with stress relaxation relative to elastic substrates. Greater spreading on substrates with stress relaxation is observed for all conditions at low substrate stiffness. Full size image Cell adhesion substrates with and without stress relaxation In order to test the predictions of the model, we investigated cell spreading on alginate substrates with and without stress relaxation. Alginate is a polysaccharide derived from seaweed. It presents no intrinsic integrin-binding sites and minimal protein absorption; however, cell adhesion can be promoted through covalent coupling of the RGD (Arg-Gly-Asp) cell adhesion peptide [22] . RGD-coupled alginate can be crosslinked into a hydrogel and used as a substrate for cell adhesion and spreading [23] . While recent work has highlighted the impact of the mode of ECM molecule tethering to substrates on cell behaviour [10] , the use of short adhesion peptides covalently coupled to the substrate avoids this potential complication as the peptide attachment to the alginate is uniform and the peptides are homogenously distributed. Importantly, covalently crosslinking the alginate itself led to elastic substrates that had little stress relaxation ( Fig. 2a , Supplementary Fig. 3 ). Some stress relaxation was measured at longer timescales; however, this was previously found to be because of water migration out of the alginate gels during bulk compression, and is likely not relevant at the length scale of a cell [24] . This interpretation was confirmed by the frequency independence of the shear storage modulus ( Fig. 2b , Supplementary Fig. 3 ). Alternatively, crosslinking the alginate ionically, with divalent cations such as Ca 2+ , led to substrates that were viscoelastic and exhibited stress relaxation ( Fig. 2a , Supplementary Fig. 3 ) because of matrix reorganization over time [24] . This was confirmed by the frequency dependence of the shear storage modulus ( Fig. 2b ), and occurs because ionic crosslinks are reversible, and can unbind and rebind when stresses are applied to the hydrogels [24] . Crosslinking was adjusted so that the initial Young’s moduli of the covalently and ionically crosslinked hydrogels, as measured by atomic force microscope indentation, could be matched for various values ( Fig. 2c ). 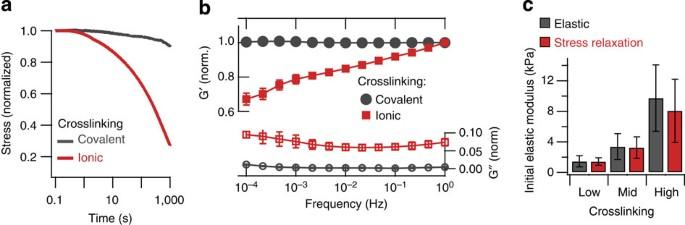Figure 2: Crosslinking alginate gels covalently or ionically lead to substrates that are either purely elastic or exhibit stress relaxation, respectively. (a) Stress relaxation of covalently and ionically crosslinked alginate gels. Covalent crosslinking led to elastic gels that show little stress relaxation. Ionically crosslinked gels were viscoelastic and exhibited stress relaxation over time under a constant strain. (b) Shear storage and shear loss modulus as a function of frequency for ionically and covalently crosslinked gels. All values are normalized by the shear storage modulus at 1 Hz for that gel. Data are shown as mean±s.d.,n=3 for each data point. (c) Initial Young’s modulus of covalently (elastic) or ionically (stress relaxing) crosslinked alginate gels as measured with atomic force microscopy for different concentrations of crosslinker (seeSupplementary Table 1). Data are shown as mean±s.d.,n=3 independent gels tested for each measurement. Figure 2: Crosslinking alginate gels covalently or ionically lead to substrates that are either purely elastic or exhibit stress relaxation, respectively. ( a ) Stress relaxation of covalently and ionically crosslinked alginate gels. Covalent crosslinking led to elastic gels that show little stress relaxation. Ionically crosslinked gels were viscoelastic and exhibited stress relaxation over time under a constant strain. ( b ) Shear storage and shear loss modulus as a function of frequency for ionically and covalently crosslinked gels. All values are normalized by the shear storage modulus at 1 Hz for that gel. Data are shown as mean±s.d., n =3 for each data point. ( c ) Initial Young’s modulus of covalently (elastic) or ionically (stress relaxing) crosslinked alginate gels as measured with atomic force microscopy for different concentrations of crosslinker (see Supplementary Table 1 ). Data are shown as mean±s.d., n =3 independent gels tested for each measurement. Full size image Substrate stress relaxation regulates cell spreading With these sets of substrates, U2OS cells were plated on substrates with various, matched initial elasticities that were crosslinked ionically or covalently. These studies revealed that the cell-spreading area increased as the initial Young’s modulus was increased from 1.4 to 9 kPa on both ionically and covalently crosslinked gels ( Fig. 3a,b , Spearman’s rank correlation P <0.001), consistent with previous work and our simulations. Interestingly, at a low modulus of 1.4 kPa greater cell-spreading area and stress fibre formation were observed on substrates that exhibit stress relaxation compared with purely elastic substrates, consistent with the model prediction. Strikingly, this effect was enhanced as ligand density was increased (Spearman’s rank correlation, P <0.0001), as cell spreading increased monotonically as a function of increased ligand density on substrates that exhibit stress relaxation ( Fig. 3c,d ). In contrast, as the ligand density was increased on purely elastic substrates, a slight increase in cell spreading was observed at intermediate ligand densities, followed by a decrease in cell spreading at higher ligand densities, consistent with previous results [6] ( Fig. 3c,d ). At high ligand densities, greater cell focal adhesion formation was observed, as indicated by the punctate localization of paxillin, on substrates with stress relaxation compared to purely elastic substrates ( Fig. 3d ). In addition, the number of cells that formed stress fibres increased significantly on substrates that exhibited stress relaxation relative to elastic substrates ( Fig. 3e ). Similarly, enhanced cell spreading on stress-relaxing substrates relative to elastic substrates at lower elasticities and higher ligand densities was found for spreading of 3T3 mouse fibroblasts ( Supplementary Fig. 4 ). While recent work has proposed a connection between the ratio of G′ to G′′ and movement of epithelial cell sheets [25] , no correlation between G′′ or the ratio of G′/G′′ with cell spreading was found here ( Supplementary Fig. 5 ). 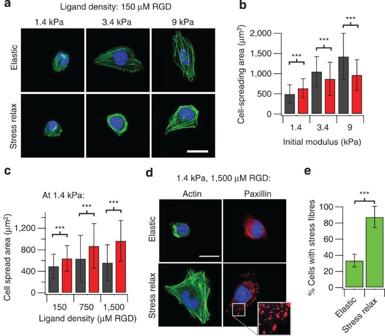Figure 3: Cell spreading enhanced for cells on substrates that exhibit stress relaxation at a low initial elasticity and high ligand density. (a) Representative images of cells plated on the indicated conditions, taken after 20 h. Actin is depicted in green; the nucleus is depicted in blue. (b) Quantification of the cell-spreading area as a function of initial modulus for cells on elastic (grey) or stress-relaxing (maroon) substrates with RGD density 150 μM.n=38–81 cells analysed for each data point. (c) Quantification of the cell-spreading area as a function of RGD ligand density for cells on elastic (grey) or stress-relaxing (maroon) substrates. The initial modulus is 1.4 kPa for all substrates.n=61–108 cells analysed for each condition. (d) Representative image of cells plated on substrates with an initial modulus of 1.4 kPa, RGD density 1,500 μM and the indicated stress relaxation behaviour stained for either actin or paxillin. Inset image is a zoom-in of the boxed region of the Paxillin stain of a cell on a substrate that exhibits stress relaxation. Punctate localization of paxillin indicates the formation of focal adhesions. (e) Quantification of the number of cells forming stress fibres on elastic and stress-relaxing substrates with an initial modulus of 1.4 kPa, RGD density 1,500 μM.n=5 independent gels for each condition. Data are shown as mean±s.d. for all panels, and ***P<0.001 (Student’st-test). Scale bars, 25 μm. Figure 3: Cell spreading enhanced for cells on substrates that exhibit stress relaxation at a low initial elasticity and high ligand density. ( a ) Representative images of cells plated on the indicated conditions, taken after 20 h. Actin is depicted in green; the nucleus is depicted in blue. ( b ) Quantification of the cell-spreading area as a function of initial modulus for cells on elastic (grey) or stress-relaxing (maroon) substrates with RGD density 150 μM. n =38–81 cells analysed for each data point. ( c ) Quantification of the cell-spreading area as a function of RGD ligand density for cells on elastic (grey) or stress-relaxing (maroon) substrates. The initial modulus is 1.4 kPa for all substrates. n =61–108 cells analysed for each condition. ( d ) Representative image of cells plated on substrates with an initial modulus of 1.4 kPa, RGD density 1,500 μM and the indicated stress relaxation behaviour stained for either actin or paxillin. Inset image is a zoom-in of the boxed region of the Paxillin stain of a cell on a substrate that exhibits stress relaxation. Punctate localization of paxillin indicates the formation of focal adhesions. ( e ) Quantification of the number of cells forming stress fibres on elastic and stress-relaxing substrates with an initial modulus of 1.4 kPa, RGD density 1,500 μM. n =5 independent gels for each condition. Data are shown as mean±s.d. for all panels, and *** P <0.001 (Student’s t -test). Scale bars, 25 μm. Full size image Next, the mechanistic basis for enhanced cell spreading on soft stress-relaxing substrates relative to elastic substrates at low elasticities and high ligand densities was investigated. While the ligand density was the same for elastic and stress-relaxing substrates since the same concentrations of RGD-alginate were used, it is in principle possible that the different modes of crosslinking might alter ligand presentation or accessibility. To test the possibility that RGD ligand presentation or accessibility is altered between elastic and stress-relaxing substrates, cell adhesion studies were performed on soft gels at high ligand densities. Any difference in ligand accessibility would be expected to result in a difference in cell adhesion. No difference in the percentage of U2OS cells adhered to relaxing versus elastic substrates was found, indicating that RGD presentation is similar between the substrates ( Fig. 4a ). Next, U2OS cell spreading on soft stress-relaxing substrates with a high ligand density in the presence of various pharmacological inhibitors and blocking antibodies to mechanotransduction pathways was assessed. Cell spreading was significantly reduced in the presence of a β1 integrin-blocking antibody, inhibitors of myosin-based contractility (blebbistatin for myosin II ATPase, ML-7 for myosin light chain kinase), Rho-associated kinase (Y-27632) and actin polymerization (Cytochalasin D; Fig. 4b ). These experiments together suggest that enhanced cell spreading on substrates with stress relaxation relative to purely elastic substrates at low elastic moduli and high ligand density is mediated through β1 integrin, actin polymerization and actomyosin-based contractility. This is consistent with the proposed model ( Fig. 1a ). Further, substrate stress relaxation led to increased nuclear translocation of the YAP transcriptional regulator ( Fig. 4c,d ), which is known to be the key transcriptional element mediating mechanotransduction for cells on 2D substrates [9] . Consistent with the result of enhanced nuclear translocation of YAP, proliferation is increased in this cancer cell line with substrate stress relaxation ( Fig. 4e ). Surprisingly, these findings demonstrate that cells are not simply integrating the modulus over time on substrates that exhibit stress relaxation. While it is currently thought that cell spreading and proliferation is suppressed on soft substrates, these results show unambiguously that substrate stress relaxation can directly compensate for the effect of decreased stiffness, as the effect of stress relaxation is mediated through some of the same pathways as stiffness: integrin adhesions, Rho activation, actomyosin-based contractility and nuclear translocation of YAP. 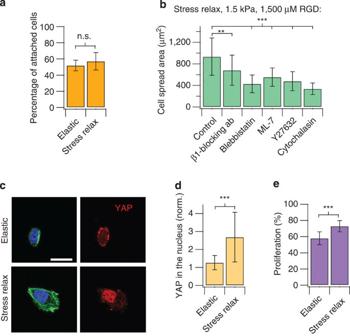Figure 4: Enhanced cell spreading on substrates with stress relaxation at a low initial elasticity is mediated through β1 integrin, actin polymerization and actomyosin contractility and is associated with increased YAP nuclear localization and proliferation. (a) Quantification of the percentage of cells adhered to stress-relaxing or elastic substrates (1.4 kPa, 1,500 μM RGD) after 20 min.n=5 gels, n.s. indicates that difference is not statistically significant by Student’st-test. (b) Quantification of the cell-spreading area on substrates with stress relaxation (initial Young’s modulus of 1.4 kPa and RGD density of 1,500 μM), with and without the addition of a β1 integrin-blocking antibody, a myosin inhibitor (blebbistatin or ML-7), a ROCK inhibitor (Y-27632) and an inhibitor of actin polymerization (Cytochalasin D).n=11–88 cells from three to four gels analysed for each condition. (c) Immunohistochemical stains of actin (green), nucleus (blue) and YAP (red) for cells on purely elastic or stress-relaxing substrates with an initial Young’s modulus of 1.4 kPa, and a RGD density of 1,500 μM. Scale bar, 25 μm. (d) Quantification of the ratio of nuclear YAP to cytoplasmic YAP for cells on substrates with an initial modulus of 1.4 kPa, and a RGD density of 1,500 μM.n=20–25 cells analysed for each condition. (e) Quantification of proliferating cells after 20 h in culture for cells on substrates with an initial modulus of 1.4 kPa and a RGD density of 1,500 μM.n≥26. Data are all shown as mean±s.d. **P<0.01 and ***P<0.001 (Student’st-test). Figure 4: Enhanced cell spreading on substrates with stress relaxation at a low initial elasticity is mediated through β1 integrin, actin polymerization and actomyosin contractility and is associated with increased YAP nuclear localization and proliferation. ( a ) Quantification of the percentage of cells adhered to stress-relaxing or elastic substrates (1.4 kPa, 1,500 μM RGD) after 20 min. n =5 gels, n.s. indicates that difference is not statistically significant by Student’s t -test. ( b ) Quantification of the cell-spreading area on substrates with stress relaxation (initial Young’s modulus of 1.4 kPa and RGD density of 1,500 μM), with and without the addition of a β1 integrin-blocking antibody, a myosin inhibitor (blebbistatin or ML-7), a ROCK inhibitor (Y-27632) and an inhibitor of actin polymerization (Cytochalasin D). n =11–88 cells from three to four gels analysed for each condition. ( c ) Immunohistochemical stains of actin (green), nucleus (blue) and YAP (red) for cells on purely elastic or stress-relaxing substrates with an initial Young’s modulus of 1.4 kPa, and a RGD density of 1,500 μM. Scale bar, 25 μm. ( d ) Quantification of the ratio of nuclear YAP to cytoplasmic YAP for cells on substrates with an initial modulus of 1.4 kPa, and a RGD density of 1,500 μM. n =20–25 cells analysed for each condition. ( e ) Quantification of proliferating cells after 20 h in culture for cells on substrates with an initial modulus of 1.4 kPa and a RGD density of 1,500 μM. n ≥26. Data are all shown as mean±s.d. ** P <0.01 and *** P <0.001 (Student’s t -test). Full size image As cell traction forces will be relaxed by matrix reorganization and flow on substrates that exhibit stress relaxation, local matrix remodelling was examined both computationally and experimentally. Alteration of node spacing on substrates with stress relaxation was compared with node spacing on purely elastic substrates in the computational model. Substrate flow and plastic deformation were found to be associated with cell spreading on substrates that exhibit stress relaxation, but not with purely elastic substrates ( Fig. 5a,b ). While the density of RGD-alginate on the ionically crosslinked substrates is initially uniform, local clustering of RGD alginate by cells has been reported previously [23] , and here was found to be greater than clustering of RGD alginate on covalently crosslinked substrates ( Supplementary Fig. 6 ). These findings indicate that enhanced cell spreading on substrates that exhibit stress relaxation is associated with local substrate remodelling. 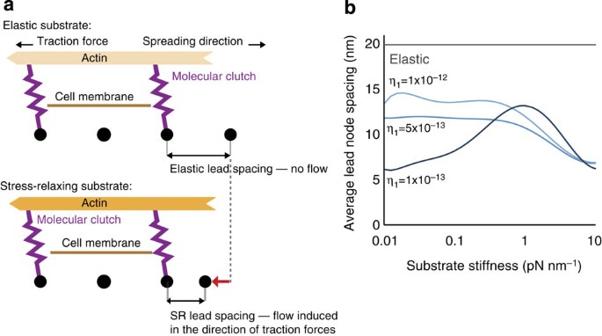Figure 5: Simulations predict that cell spreading on stress-relaxing substrates is associated with flow and plastic deformation of the adhesion substrate. (a) Cartoon of cell spreading on elastic substrate or substrate with stress relaxation. (b) Simulation results for lead node spacing as a function of substrate stiffness for elastic substrates, and stress-relaxing substrates with the indicated Burger’s model Maxwell damping coefficient (η1). Figure 5: Simulations predict that cell spreading on stress-relaxing substrates is associated with flow and plastic deformation of the adhesion substrate. ( a ) Cartoon of cell spreading on elastic substrate or substrate with stress relaxation. ( b ) Simulation results for lead node spacing as a function of substrate stiffness for elastic substrates, and stress-relaxing substrates with the indicated Burger’s model Maxwell damping coefficient ( η 1 ). Full size image Taken together, these findings indicate that parallel to stiffness, substrate stress relaxation is a fundamental physical property of model ECM that has a substantial impact on cell behaviour and function. The effect of stress relaxation was mediated through integrin adhesions and actomyosin-based contractility, and increased stress relaxation drives nuclear translocation of YAP. This suggests that increased stress relaxation can compensate for matrices with a lower stiffness. Consistent with this idea, cell spreading and proliferation were increased on substrates with stress relaxation, compared with elastic substrates with the same initial elastic modulus. Reorganization of the actin cytoskeleton in response to mechanical cues initiates within seconds [3] , and, in the case of cell spreading, equilibrates over minutes to hours [26] , which is consistent with cells responding to stress relaxation on the order of minutes as observed here ( Fig. 2a ). Previous studies with cells cultured on purely elastic substrates have found that the stored elastic energy increases with the substrate modulus because of an increase in cellular traction stress [4] , [27] ; however, it is unclear how this translates to viscoelastic substrates. One possibility is that the dissipation of energy through matrix yielding, and resultant decrease in stored energy, allows cells to generate more work on viscoelastic substrates relative to purely elastic substrates of the same elasticity, and this may enable spreading. Indeed, the computational model predicts and experiments find that substrate flow and plastic deformation are associated with cell spreading on substrates that exhibit stress relaxation ( Fig. 5a,b ). Since RGD clustering is known to influence cell adhesion and spreading and promote integrin signalling, the ability to mechanically cluster ligands by cells on stress-relaxing substrates may activate spreading behaviours in the cells [28] , [29] . Generally, the findings of our computational model suggest that this behaviour may be an intrinsic, yet unexpected, result of molecular clutch-based adhesions. A recent study showed that an increase in the loss modulus of polyacrylamide substrates led to increased cell spreading as well [12] . However, because of the covalent crosslinking and an associated time-independent storage modulus of these substrates, as well as possible alterations in pore size arising from the method used to modulate the loss modulus [10] , it is likely that the mechanism for enhanced cell spreading differs in that study. Interestingly, our results might in part explain why high cell spreading was observed on soft but highly stress-relaxing polydimethylsiloxane (PDMS) substrates in a recent paper [10] . Overall, our results show that the hypothesis that mechanotransduction is solely mediated through cells sensing resistance to traction forces does not hold for cells on soft viscoelastic substrates. Since physiological extracellular matrices typically exhibit various degrees of stress relaxation, this finding highlights the importance of considering matrix stress relaxation as a fundamental property of the ECM that is critical to understand the basics of cell–ECM interactions and the underlying biophysics of mechanotransduction. Alginate preparation Sodium alginate rich in guluronic acid blocks and with a high molecular weight (280 kDa, LF20/40) was purchased from FMC Biopolymer. RGD alginate was prepared by coupling the oligopeptide GGGGRGDSP (Peptides International) to the alginate using standard carbodiimide chemistry. In a typical reaction, 1 g of alginate was reconstituted at 1% wt/vol in MES Buffer (0.1 M MES, 0.3 M NaCl, pH 6.5). For the highest ligand density, RGD alginate used in this study (corresponding to 1,500 μM RGD condition), 274 mg of sulfo-NHS (Pierce), 484 mg of N-(3-Dimethylaminopropyl)-N'-ethylcarbodiimide (EDC) (Sigma) and 112 mg of GGGGRGDSP peptide were added, and the reaction was allowed to proceed for 20 h. For synthesis of RGD alginate with other ligand densities, the quantities of sulfo-NHS, EDC and RGD peptide were scaled accordingly. Concentrations of RGD were chosen such that 2, 10 or 20 RGD peptides were coupled to one alginate chain on average [22] . These correspond to densities of 150, 750 and 1,500 μM RGD in a 2% wt/vol alginate gel. Alginate was dialysed against deionized water for 2–3 days (molecular weight cutoff of 3.5 kDa), filtered with activated charcoal, sterile-filtered, lyophilized and then reconstituted in serum-free DMEM (Dulbecco’s Modified Eagles Medium, Life Technologies) for ionic crosslinking, or MES buffer for covalent crosslinking. Mechanical characterization Atomic force microscopy (AFM) measurements of the Young’s modulus of the alginate gels were performed with an MFP-3D system (Asylum Research) using silicon nitride cantilevers (MLCT, Bruker AFM Probes). The stiffness was calibrated from the thermal fluctuations of the cantilever in air, and cantilevers with a stiffness of ~13 pN nm −1 were used. The cantilever was moved towards the stage at a rate of 1 μm s −1 and force indentation curves were interpreted using the Hertzian model for a pyramidal indentor [30] . Rheology measurements were made with an AR-G2 stress-controlled rheometer (TA Instruments). Alginate gels were deposited directly on the surface plate of the rheometer immediately after mixing with the crosslinker. A 20 mm plate was immediately brought down, forming a 20 mm disk of gel with an average thickness of ~1.8 mm. The mechanical properties were then measured over time until the storage modulus reached an equilibrium value. The storage modulus at 0.5% strain and at 1 Hz was recorded periodically until the storage modulus reached its equilibrium value. Then, a strain sweep was performed to confirm that this value was within the linear elastic regime, followed by a frequency sweep. No prestress was applied to the gels for these measurements. The stress relaxation properties of alginate gels were also measured from compression tests of the gel disks (15 mm in diameter, 2 mm thick, equilibrated in DMEM for 24 h) [24] , [31] . The gel disks were compressed to 15% strain with a deformation rate of 1 mm min −1 using an Instron 3342 single-column mechanical tester. Subsequently, the strain was held constant, while the load was recorded as a function of time. Cell culture U2OS and 3T3 fibroblasts (ATCC) were cultured in standard DMEM (Invitrogen) with 10% fetal bovine serum (Invitrogen) and 1% penicillin/streptomycin (Invitrogen). Plating of cells on gels One-millimetre-thick alginate hydrogels were prepared [24] , [31] . Briefly, for ionically crosslinked gels, 0.8 ml RGD alginate in serum-free DMEM was rapidly mixed with 0.2 ml DMEM containing the appropriate amount of calcium sulfate (final concentrations detailed in Supplementary Table 1 ) using luerlock syringes (Cole-Parmer) and a female–female luerlock coupler (Value plastics). Then, the mixed solution was quickly deposited between two glass plates spaced 1 mm apart. The solution was allowed to gel for 2 h. For covalently crosslinked gels, 0.8 ml RGD alginate in MES buffer was mixed with 0.2 ml MES buffer containing 2.5 mg ml −1 of 1-Hydroxybenzotriazole (HOBt, from Sigma), 50 mg ml −1 EDC and the appropriate amount of adipic acid dihydrazide (AAD from Sigma, final concentrations detailed in Supplementary Table 1 ). Then, the mixed solution was quickly deposited between two glass plates spaced 1 mm apart. The solution was allowed to gel for 12 h. Following gelation, 15 mm disks were punched out, and these disks were washed thoroughly four times over 2 days in serum-free media. Disks were held at the bottom of a well plate by a customized plastic insert (so that they did not float when submerged in media), and the cells were plated at a low density of 10,000 cells cm −2 , so that they did not contact other cells on average. Cells were allowed to spread for 20 h, and then were fixed and stained for analysis. Only isolated cells, without any cell–cell contacts, were analysed. Immunohistochemistry For immunohistochemical staining, media were first removed from the gels. The gels were then fixed with 4% paraformaldehyde in serum-free DMEM at 37 °C for 30–45 min. Gels were then washed three times in PBS containing calcium (cPBS). Gels were stained following standard immunohistochemistry protocols directly after washing. The following antibodies/reagents were used for immunohistochemistry: YAP antibody (Cell signaling, Catalogue no. 4912, dilution of 1:100), Paxillin antibody (Abcam, Catalogue no. ab32084, dilution of 1:200), Prolong Gold antifade reagent with 4',6-diamidino-2-phenylindole (DAPI; Invitrogen), AF-488 Phalloidin to stain actin (Life Technologies, dilution of 1:80), Goat anti-Rabbit IgG AF 647 (Invitrogen, Catalogue no. a21245, dilution of 1:500). The Click-IT EdU cell proliferation assay (Invitrogen) was used to identify proliferating cells. Image analysis For measurements of the cell-spreading area in 2D, images of phalloidin/DAPI-stained cells were taken for the indicated conditions at × 20 or × 63 with a laser scanning confocal microscope (LSM 710, Zeiss). Only those cells that did not exhibit any cell–cell contacts were considered in the analysis. Images of all single cells were then thresholded manually on the basis of the actin stain, and the area of the thresholded cell body was determined using a custom macro in ImageJ (NIH). For measurements of YAP nuclear localization, images of DAPI/phalloidin/YAP antibody-stained cells were taken with an NA=1.40 63X PlanApo oil immersion objective with a LSM. Images were thresholded on each colour channel to determine the nuclear area and cell/cytoskeleton area outside of the nucleus. The YAP nuclear localization ratio was then determined as the summed intensity of the YAP signal within the nucleus normalized by the nuclear area divided by the summed intensity of the YAP signal outside of the nucleus normalized by the non-nuclear cytoskeleton area. Blocking antibody and inhibitor experiments Cells were plated on hydrogel substrates at a density of 10,000 cells cm −2 . Cells were allowed to spread for 20 h at the presence of one of the following reagents: β1 integrin blocking antibody (5 μg ml −1 or dilution of 1:200, clone P5D2, EMD Millipore, Catalogue no. MAB1959), blebbistatin (50 μM, Tocris Bioscience), ML-7 hydrochloride (25 μM, Tocris Bioscience), Y-27632 dihydrochloride (10 μM, Tocris Bioscience) or cytochalasin D (2 μM, Sigma-Aldrich). The cells were then fixed and stained for analysis. Only isolated cells, without any cell–cell contacts, were analysed. Cell adhesion experiments Cells were plated on hydrogel substrates at a density of 20,000 cells cm −2 . Cells were allowed to adhere for 20 min at 37 °C in a tissue culture incubator. All the media were then collected and the cells that did not adhere to the substrates were counted immediately with an automated cell counter (Countess cell counter, Life Technologies). The adhered cells were calculated by subtracting non-adhered cells from the total number of cells for each experiment. RGD-clustering experiments Tetramethylrhodamine (TAMRA)-labelled RGD peptide (GGGGRGDSPASSK-TAMRA, Peptides International) was coupled to alginate [23] , [31] . TAMRA-labelled RGD alginate was mixed with non-labelled RGD alginate at a ratio of 1:9 or 1:19 before crosslinking; therefore, the resulting hydrogel substrates have a fraction of fluorescently labelled RGD uniformly distributed in the gels. Cells were plated at a density of 10,000 cells cm −2 and were allowed to spread for 40 h. Cells were then imaged live on the substrates with a confocal microscope. How to cite this article: Chaudhuri, O. et al . Substrate stress relaxation regulates cell spreading. Nat. Commun. 6:6365 doi: 10.1038/ncomms7365 (2015).